Thymic epithelial cell expansion through matricellular protein CYR61 boosts progenitor homing and T-cell output Thymic epithelial cells (TEC) are heterogeneous stromal cells that generate microenvironments required for the formation of T cells within the thymus. Defects in TEC lead to immunodeficiency or autoimmunity. Here we identify TEC as the major source of cysteine-rich protein 61 (CYR61), a matricellular protein implicated in cell proliferation and migration. Binding of CYR61 to LFA-1, ICAM-1 and integrin α6 supports the adhesion of TEC and thymocytes as well as their interaction. Treatment of thymic lobes with recombinant CYR61 expands the stromal compartment by inducing the proliferation of TEC and activates Akt signalling. Engraftment of CYR61-overexpressing thymic lobes into athymic nude mice drastically boosts the yield of thymic output via expansion of TEC. This increases the space for the recruitment of circulating hematopoietic progenitors and the development of T cells. Our discovery paves the way for therapeutic interventions designed to restore thymus stroma and T-cell generation. Hematopoietic progenitor cells recruited from the blood to the thymus embrace a T-cell lineage fate within specific microenvironments created by stromal cells [1] , [2] , [3] . Thymic epithelial cells (TEC) are the main stromal cell population and orchestrate the migration, proliferation and survival of differentiating thymocytes. TEC are subdivided into cortical TEC (cTEC) and medullary TEC (mTEC), with different localization and functions [2] , [4] , [5] . A decrease in the number of TEC and a compromised medullary and cortical architecture are characteristics of age-associated thymic involution. The resulting decrease in T-cell production ensues in a loss of repertoire diversity. Similarly, cytoablative treatments also severely impair thymic structure and function [6] . Deciphering the molecular mechanisms underlying TEC function and the formation of thymic microenvironments is mandatory for the development of therapies. To date, cytokines of the TNF superfamily, such as RANKL, CD40L and lymphotoxin, have been reported to promote the development and maturation of mTEC [7] , whereas Keratin Growth Factor (KGF) has been implicated in thymic regeneration [8] . In addition, thymic innate lymphoid cell-derived IL-22 has been reported recently to participate in endogenous thymic regeneration by inducing TEC proliferation [9] . Components of the extracellular matrix (ECM) are critically involved in the formation of thymic microenvironments. They constitute molecular bridges between thymocytes and stromal cells, supporting migration and development of thymocytes and TEC [10] , [11] , [12] , [13] . CYR61 (CYsteine-Rich protein 61) is an ECM cell adhesive protein produced by several cells, including endothelial cells, fibroblasts and smooth muscle cells [14] . CYR61 has been implicated in carcinogenesis, wound healing and cardiovascular development through binding to integrins such as αVβ3, αMβ2 and α6β1 (refs 14 , 15 , 16 , 17 ). Notably, Cyr61 -deficient mice are embryonic lethal because of cardiovascular defects [18] . Depending on the cell type and context, CYR61 can promote the proliferation, survival, migration or senescence of cells [14] , [17] , [18] , [19] , [20] . CYR61 is overexpressed in various cancer cells, including cancers of epithelial origin, and can promote their proliferation [21] , [22] , [23] . Furthermore, specific expression of CYR61 in thymic stroma was evidenced in a study aimed at mapping thymic stromal gene expression [24] . However, the role of CYR61 in the thymus has not been addressed previously. As CYR61 promotes cell proliferation [14] , [16] , [21] , we examine here the benefits of CYR61 treatment on T-cell development and the thymic stroma. We observe that matricellular protein CYR61 specifically induces the proliferation of TEC and the expansion thymic stroma in vitro . In vivo , engraftment of thymic lobes that modestly overexpress CYR61 dramatically boosts the production of T cells in athymic nude mice via the expansion of TEC. Detailed analyses reveal that the stromal expansion induced by CYR61 creates additional space for the recruitment of circulating hematopoietic progenitors and for the development of T cells. Importantly, animals grafted with CYR61-overexpressing thymus display a normal T-cell repertoire without any signs of autoimmunity. Our results show that CYR61 treatment increases the size of the thymus via expansion of TEC, thus enabling the recruitment of circulating progenitors and the production of T cells. TEC are the main source of CYR61 in the thymus We first quantified the expression of CYR61 in different thymic cell populations in adult mice. Quantitative PCR revealed CYR61 expression in TEC, fibroblasts and endothelial cells ( Fig. 1a ). We then investigated CYR61 expression at the protein level. Intracellular staining of CYR61 protein detected by flow cytometry revealed higher expression in cTEC (EpCAM + ,CD45 neg ,Ly51 + ) and mTEC (EpCAM + ,CD45 neg ,Ly51 −/low ) compared with the other populations ( Fig. 1b ). Some protein expression was also detected in the CD45 neg ,EpCAM neg population that comprises fibroblasts and endothelial cells but at a far lesser extent than in TEC ( Fig. 1b ). No CYR61 was detected on cell surface according to FACS analyses on non-permeabilized cells ( Supplementary Fig. S1a ). Finally, CYR61 production by TEC was further confirmed with thymic sections stained for the mTEC marker keratin 5 (K5) and cTEC marker keratin 8 (K8) ( Fig. 1c ). Control staining for CYR61 is provided in Supplementary Fig. S1b . Hence, TEC are the main source of CYR61 in the thymus. 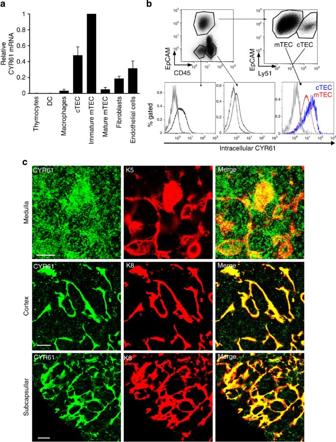Figure 1: TEC are the main source of CYR61 in the thymus. (a) Adult murine thymus. mRNA expression of CYR61 measured by qRT–PCR in thymocytes, DC (CD45+, CD11chigh), macrophages (CD45+, F4/80+), cTEC (CD45neg, EpCAM+, Ly51+), immature mTEC (CD45neg, EpCAM+, Ly51−/low, CD80−), mature mTEC (CD45neg, EpCAM+, Ly51−/low, CD80high), fibroblasts (CD45neg, PDGFRα+) and endothelial cells (CD45neg, PECAM+). Expression was normalized to immature mTEC and represents the mean ±s.d. of two to four independent experiments. (b) Flow cytometry profile for intracellular CYR61 expression of CD45+-depleted thymic cells of adult murine thymus. (c) Thymic sections from adult mice were stained for CYR61, K5 (mTEC marker) and K8 (cTEC marker) expression. Scale bars, 10 μm. Control staining for CYR61 is provided inSupplementary Fig. S1b. Figure 1: TEC are the main source of CYR61 in the thymus. ( a ) Adult murine thymus. mRNA expression of CYR61 measured by qRT–PCR in thymocytes, DC (CD45 + , CD11c high ), macrophages (CD45 + , F4/80 + ), cTEC (CD45 neg , EpCAM + , Ly51 + ), immature mTEC (CD45 neg , EpCAM + , Ly51 −/low , CD80 − ), mature mTEC (CD45 neg , EpCAM + , Ly51 −/low , CD80 high ), fibroblasts (CD45 neg , PDGFRα + ) and endothelial cells (CD45 neg , PECAM + ). Expression was normalized to immature mTEC and represents the mean ±s.d. of two to four independent experiments. ( b ) Flow cytometry profile for intracellular CYR61 expression of CD45 + -depleted thymic cells of adult murine thymus. ( c ) Thymic sections from adult mice were stained for CYR61, K5 (mTEC marker) and K8 (cTEC marker) expression. Scale bars, 10 μm. Control staining for CYR61 is provided in Supplementary Fig. S1b . Full size image Binding to CYR61 enhances TEC interactions with thymocytes As CYR61 is a secreted molecule with cell adhesive properties [14] , we wondered whether CYR61 can support the adhesion of thymocytes or TEC. Thymocytes, primary TEC and IT76M1, a mouse TEC cell line, were seeded on microplates coated with recombinant CYR61-Fc protein or Fc molecule. As shown in Fig. 2a and Supplementary Fig. S2a , CYR61 was able to support the adhesion of both thymocytes and TEC. 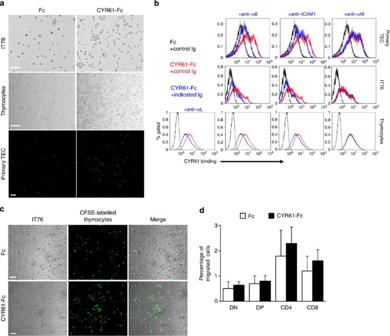Figure 2: CYR61 binding enhances TEC/thymocyte interactions. (a) Microtiter wells were coated with recombinant CYR61-Fc (5 μg ml−1) or Fc molecule. IT76 or thymocytes were seeded in serum-free medium and incubated at 37 °C for 90 min. Data are representative of three experiments. Primary TEC-enriched cell suspensions were labelled with FITC-coupled anti-EpCAM antibody then seeded in serum-free medium and incubated at 37 °C for 60 min. Data are representative of four preparations. Quantifications are provided inSupplementary Fig. S2a. Scale bars, 100 μm. (b) Binding of CYR61 (1 μg ml−1) was assessed by flow cytometry. Primary TEC, IT76 or thymocytes were preincubated with control rabbit Ig or polyclonal rabbit antibodies (50 μg ml−1) against integrin α6, αL, αM or ICAM1 for 45 min at RT. Cells were treated with recombinant Fc or CYR61-Fc for 15 min at RT. CYR61 binding was detected by flow cytometry using an AF488-coupled anti-human Fc antibody. In the case of primary TEC, recombinant Fc and CYR61-Fc were directly coupled to DyLight 650 and CYR61 binding was assessed by FACS gated on EpCAM+,CD45negTEC cells. Data are representative of three experiments. Quantification is provided inSupplementary Fig. S2b. (c) Adhesion of CFSE-labelled thymocytes on IT76M1 monolayers pretreated with CYR61-Fc (5 μg ml−1) or Fc molecules at 37 °C for 60 min. Data are representative of three experiments. Quantification is provided inSupplementary Fig. S2c. Scale bars, 100 μm. (d) Chemotaxis assay. Migration of thymocytes toward CYR61-Fc (5 μg ml−1) or Fc molecule using transwell cell migration chambers. Migration after 3 h is provided as a percentage of migrated subsets of thymocytes±s.e.m. (n=4). Figure 2: CYR61 binding enhances TEC/thymocyte interactions. ( a ) Microtiter wells were coated with recombinant CYR61-Fc (5 μg ml −1 ) or Fc molecule. IT76 or thymocytes were seeded in serum-free medium and incubated at 37 °C for 90 min. Data are representative of three experiments. Primary TEC-enriched cell suspensions were labelled with FITC-coupled anti-EpCAM antibody then seeded in serum-free medium and incubated at 37 °C for 60 min. Data are representative of four preparations. Quantifications are provided in Supplementary Fig. S2a . Scale bars, 100 μm. ( b ) Binding of CYR61 (1 μg ml −1 ) was assessed by flow cytometry. Primary TEC, IT76 or thymocytes were preincubated with control rabbit Ig or polyclonal rabbit antibodies (50 μg ml −1 ) against integrin α6, αL, αM or ICAM1 for 45 min at RT. Cells were treated with recombinant Fc or CYR61-Fc for 15 min at RT. CYR61 binding was detected by flow cytometry using an AF488-coupled anti-human Fc antibody. In the case of primary TEC, recombinant Fc and CYR61-Fc were directly coupled to DyLight 650 and CYR61 binding was assessed by FACS gated on EpCAM + ,CD45 neg TEC cells. Data are representative of three experiments. Quantification is provided in Supplementary Fig. S2b . ( c ) Adhesion of CFSE-labelled thymocytes on IT76M1 monolayers pretreated with CYR61-Fc (5 μg ml −1 ) or Fc molecules at 37 °C for 60 min. Data are representative of three experiments. Quantification is provided in Supplementary Fig. S2c . Scale bars, 100 μm. ( d ) Chemotaxis assay. Migration of thymocytes toward CYR61-Fc (5 μg ml −1 ) or Fc molecule using transwell cell migration chambers. Migration after 3 h is provided as a percentage of migrated subsets of thymocytes±s.e.m. ( n =4). Full size image CYR61 binds to various molecules on the cell surface including integrins αM and α6 (refs 15 , 16 , 17 ). Blocking integrin α6 and ICAM1 with antibodies inhibited CYR61 binding to IT76M1, primary TEC and thymocytes ( Fig. 2b , Supplementary Fig. S2b ). Meanwhile, targeting CD11b (integrin αM), which is not expressed in TEC and thymocytes, was ineffective ( Fig. 2b ). In the case of thymocytes, blocking CD11a (integrin αL) also inhibited CYR61 binding ( Fig. 2b , Supplementary Fig. S2b ). T-cell development relies on interactions between thymocytes and TEC [25] , while the ECM provides a structural support for cell migration and adhesion [10] . In addition, TEC and thymocytes interact through molecules such as LFA1/ICAM1 (refs 25 , 26 ). To test whether CYR61 would affect such interactions, adhesion of CFSE-labelled thymocytes to monolayers of IT76M1 pretreated either with CYR61-Fc or Fc molecule for 1 h was assayed. We observed that CYR61 increased adhesion of thymocytes to TEC monolayers ( Fig. 2c , Supplementary Fig. S2c ). Although CYR61 can promote or inhibit cell migration depending on cell type [19] , [20] , we observed no chemotactic activity of CYR61 on any thymocyte subset ( Fig. 2d ). We conclude that CYR61 binds to ICAM1 and integrin α6 on the TEC surface, but also to integrin αL on thymocytes, supporting cell adhesion and interaction. CYR61 induces TEC proliferation As CYR61 induces the proliferation of various cell types [14] , [27] , we investigated whether CYR61 treatment would promote TEC proliferation. Fetal thymic organ cultures (FTOC) were depleted of thymocytes with 2'-deoxyguanosine (2DG-FTOC). Supplementing 2DG-FTOC with recombinant CYR61 drastically increased thymic stroma size and TEC numbers ( Fig. 3a,b ). Neither relative mTEC and cTEC frequencies nor their maturation based on MHC class II expression was affected ( Supplementary Fig. S3 ). The effect was specific of TEC because the number of CD45 neg ,EpCAM neg was not modified after treatment ( Fig. 3b ). A direct effect of CYR61 on TEC was further confirmed with the mouse TEC cell line IT76M1. Treatment with CYR61 increased absolute numbers of IT76M1 ( Fig. 3c ). Accordingly, the percentage of proliferating Ki67 + cells was almost twofold higher than in controls after 72 h ( Fig. 3d ). 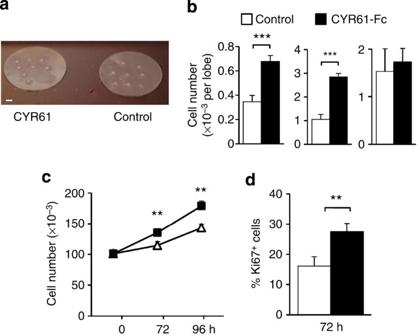Figure 3: CYR61 treatment induces TEC proliferation. (a,b) 2DG-FTOC were cultured for 4 days in the presence of CYR61-Fc. Scale bar 1 mm. Cell numbers were quantified by flow cytometry. Data±s.e.m. are representative of three independent experiments. (c) IT76M1 cells were cultured in the presence or absence of CYR61-Fc for the indicated times. Cell numbers were determined by flow cytometry. Data are the mean of three experiments ±s.e.m. (d) The percentage of proliferating Ki67+IT76M1 after 72 h of treatment with CYR61-Fc was quantified by flow cytometry. Data are the mean of two experiments±s.d. **P≤0.01; ***P≤0.001 (two-tailed unpaired Student’st-test). Figure 3: CYR61 treatment induces TEC proliferation. ( a , b ) 2DG-FTOC were cultured for 4 days in the presence of CYR61-Fc. Scale bar 1 mm. Cell numbers were quantified by flow cytometry. Data±s.e.m. are representative of three independent experiments. ( c ) IT76M1 cells were cultured in the presence or absence of CYR61-Fc for the indicated times. Cell numbers were determined by flow cytometry. Data are the mean of three experiments ±s.e.m. ( d ) The percentage of proliferating Ki67 + IT76M1 after 72 h of treatment with CYR61-Fc was quantified by flow cytometry. Data are the mean of two experiments±s.d. ** P ≤0.01; *** P ≤0.001 (two-tailed unpaired Student’s t -test). Full size image We next investigated which signalling pathways would be modulated by CYR61 treatment using the IT76M1 cell line to face the issue of highly restricted cell numbers in FTOC. CYR61 induced Akt phosphorylation in IT76M1 cells ( Fig. 4a ), whereas ERK1/2 phosphorylation was transiently repressed ( Supplementary Fig. S4 ). Analysis of NF-κB activation (through I-κB degradation), and phosphorylation of JNK and p38, excluded any implication of these pathways ( Supplementary Fig. S4 ). Previous studies showed that reduced Akt activity in TEC was responsible for altered thymic architecture, early involution and defects in keratinocyte proliferation [28] , [29] , [30] . In order to determine the implication of Akt in CYR61-mediated TEC proliferation, 2DG-FTOC were cultured with recombinant CYR61 in the presence of Akt inhibitor MK2206. Inhibition of Akt suppressed the effect of CYR61 on TEC numbers ( Fig. 4b ) as well as the blocking of integrin α6 ( Fig. 4c ). Collectively, our data show that matricellular protein CYR61-induced proliferation of TEC was thymocyte-independent and stimulated α6-integrin and the Akt signalling pathway. 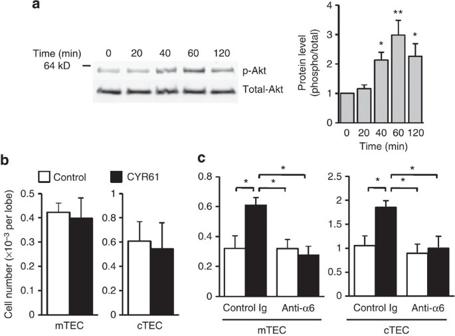Figure 4: CYR61-induced TEC proliferation is integrin α6-dependent. (a) Immunoblot analysis of phospho- and total-Akt in lysates of IT76M1 stimulated with CYR61-Fc (5 μg ml−1) for the indicated times. Data is representative of three to four experiments±s.e.m. Quantification is provided on the right. *P≤0.05; **P≤0.01 (one-way ANOVA, Dunnet test) Full blots are provided inSupplementary Fig. S8. (b,c) 2DG-FTOC were cultured for 3 days in the presence of CYR61-Fc (5 μg ml−1) and Akt inhibitor MK2206 (1 μM) (b) or anti-integrin α6 or control antibodies (50 μg ml−1) (c). Cell numbers were quantified by flow cytometry (representative of two experiments±s.d.). *P≤0.05 (two-way ANOVA, Tukey HSD test). Figure 4: CYR61-induced TEC proliferation is integrin α6-dependent. ( a ) Immunoblot analysis of phospho- and total-Akt in lysates of IT76M1 stimulated with CYR61-Fc (5 μg ml −1 ) for the indicated times. Data is representative of three to four experiments±s.e.m. Quantification is provided on the right. * P ≤0.05; ** P ≤0.01 (one-way ANOVA, Dunnet test) Full blots are provided in Supplementary Fig. S8 . ( b , c ) 2DG-FTOC were cultured for 3 days in the presence of CYR61-Fc (5 μg ml −1 ) and Akt inhibitor MK2206 (1 μM) ( b ) or anti-integrin α6 or control antibodies (50 μg ml −1 ) ( c ). Cell numbers were quantified by flow cytometry (representative of two experiments±s.d.). * P ≤0.05 (two-way ANOVA, Tukey HSD test). Full size image CYR61 enhances thymic output Integrity of thymic stroma being essential, we aimed at improving thymus function in vivo by expansion of TEC with CYR61. To this purpose, 2DG-FTOC were transduced with a lentiviral CYR61 expression vector or a control vector, and grafted under the renal capsules of B6-nude mice ( Supplementary Fig. S5a ). CYR61 expression was increased 4.5-fold ( Supplementary Fig. S5b ) with >90% of TEC being transduced, based on GFP expression ( Supplementary Fig. S5c ). Nude mice lack functional thymus and are therefore devoid of T cells because they bear a spontaneous mutation in the FoxN1 gene [31] , a transcription factor essential for TEC development [32] . As hematopoietic precursors are normal in nude, transplantation of WT-thymic lobes into nude mice re-establishes normal T-cell development [33] . Similarly, thymus transplantation in infants deficient for FoxN1 or with complete DiGeorge anomaly leads to T-cell reconstitution and to normal immune function [34] , [35] . Nude mice transplanted with CYR61-overexpressing lobes (CYR61-nude) or control lobes (control-nude) were monitored for 8 weeks. The numbers of CD8 + ( Fig. 5a ) and CD4 + T cells ( Fig. 5b ) in blood was drastically increased in CYR61-nude compared with control-nude mice. The number of T cells in blood had doubled at the end of the experiment. Interestingly, the size of ectopic thymus in CYR61-nude mice was bigger than that of controls ( Fig. 5c ). The number of TEC ( Fig. 5d ) and thymocytes ( Fig. 5e ) were increased approximately twofold in CYR61-nudes, although the subset frequency was identical ( Fig. 5f ). Importantly, no signs of autoimmunity could be detected, as spleen size ( Fig. 5c ) and weight, serum IgG levels and the frequency of mature CD4 + and CD8 + T cells in the spleen were similar in both groups ( Supplementary Fig. S5d–g ). There were also no inflammatory infiltrates in the pancreas, liver, lung or kidney of CYR61-nudes ( Supplementary Fig. S5h ). Based on TCR Vβ usage, the T-cell repertoire was identical in control and CYR61 grafts ( Fig. 5g,h ). Finally, we performed a T-cell proliferation assay using CD3/CD28 stimulation on CD8 + - and CD4 + T cells purified from spleen of control-transplanted and CYR61-nude mice. Proliferative response was similar, thus indicating that T cells from CYR61-nude mice were as competent as T cells from control-transplanted nude mice ( Fig. 5i ). These findings indicate that mild overexpression of CYR61 expands TEC and boosts thymic output. 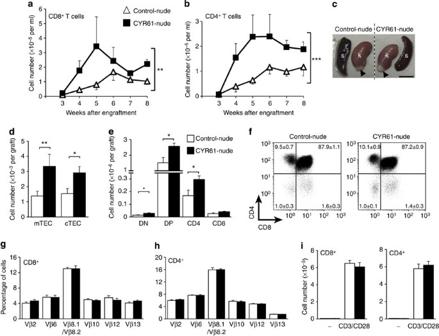Figure 5: CYR61 enhances thymic output. (a–b) Blood T-cell counts. (a) Number±s.e.m. of CD8+T cells and (b) CD4+T cells in the blood following engraftment of control-nude (n=6) and CYR61-nude mice (n=5). **P≤0.01; ***P≤0.001 (two-way ANOVA). (c) Gross anatomy of the spleen (S) and kidneys (K) 8 weeks after engraftment of thymic lobes (black arrowheads). Scale bar 10 mm. (d) Number of mTEC and cTEC±s.e.m. in grafts. *P≤0.05; **P≤0.01 (control-nude (n=6) and CYR61-nude mice (n=5), two-tailed unpaired Student’st-test). (e) Number of each thymocyte subsets±s.e.m. in grafts. *P≤0.05 (control-nude (n=6) and CYR61-nude mice (n=5), two-tailed unpaired Student’st-test). (f) CD4/CD8 distribution in grafts from control-nude and CYR61-nude mice. Percentages are mean ±s.e.m. Control-nude (n=6) and CYR61-nude mice (n=5). (g,h) Control and CYR61 lobes were grafted in each kidney of WT mice. Four weeks after transplantation, TCR Vβ usage by thymic CD4+(g) and CD8+(h) T cells were measured by FACS. Results from two independent experiments are pooled and shown ±s.e.m. (n=7). (i) T-cell proliferation assay. CD8+- and CD4+T cells from spleen were positively purified and then stimulated in anti-CD3-coated plates with anti-CD28 antibodies for 72 h. Data are the mean of control-nude (n=6) and CYR61-nude mice (n=5) ±s.e.m. Figure 5: CYR61 enhances thymic output. ( a – b ) Blood T-cell counts. ( a ) Number±s.e.m. of CD8 + T cells and ( b ) CD4 + T cells in the blood following engraftment of control-nude ( n =6) and CYR61-nude mice ( n =5). ** P ≤0.01; *** P ≤0.001 (two-way ANOVA). ( c ) Gross anatomy of the spleen (S) and kidneys (K) 8 weeks after engraftment of thymic lobes (black arrowheads). Scale bar 10 mm. ( d ) Number of mTEC and cTEC±s.e.m. in grafts. * P ≤0.05; ** P ≤0.01 (control-nude ( n =6) and CYR61-nude mice ( n =5), two-tailed unpaired Student’s t -test). ( e ) Number of each thymocyte subsets±s.e.m. in grafts. * P ≤0.05 (control-nude ( n =6) and CYR61-nude mice ( n =5), two-tailed unpaired Student’s t -test). ( f ) CD4/CD8 distribution in grafts from control-nude and CYR61-nude mice. Percentages are mean ±s.e.m. Control-nude ( n =6) and CYR61-nude mice ( n =5). ( g , h ) Control and CYR61 lobes were grafted in each kidney of WT mice. Four weeks after transplantation, TCR Vβ usage by thymic CD4 + ( g ) and CD8 + ( h ) T cells were measured by FACS. Results from two independent experiments are pooled and shown ±s.e.m. ( n =7). ( i ) T-cell proliferation assay. CD8 + - and CD4 + T cells from spleen were positively purified and then stimulated in anti-CD3-coated plates with anti-CD28 antibodies for 72 h. Data are the mean of control-nude ( n =6) and CYR61-nude mice ( n =5) ±s.e.m. Full size image CYR61 does not affect T-cell development per se Two hypotheses could account for increased thymic output. First, CYR61 could potentiate thymocyte development directly, favoring T-cell production and release. Second, CYR61-induced thymus hypertrophy could increase the hosting capacity of CYR61 lobes for circulating precursors, thus increasing T-cell development indirectly. We tested whether CYR61 directly promotes thymocyte development using FTOC. Thymic lobes are composed of a complete stromal compartment and a defined number of thymocyte precursors, which differentiate over time. Two days after treatment with recombinant CYR61, the frequency and the number of thymocyte subsets were similar to controls ( Fig. 6a,b ). After 6 days of culture, differentiation of thymocytes had progressed but still no difference was observed between CYR61-treated cultures and controls ( Fig. 6c,d ). However, recombinant CYR61 increased the number of TEC by day 2 of treatment ( Fig. 6e ), consistent with 2DG-FTOC experiments ( Fig. 3a,b ). Six days after CYR61 treatment, the number of TEC remained higher than controls but the difference did not further intensify ( Fig. 6f ). Neither the relative mTEC and cTEC frequencies nor their maturation were affected ( Supplementary Fig. S6 ). 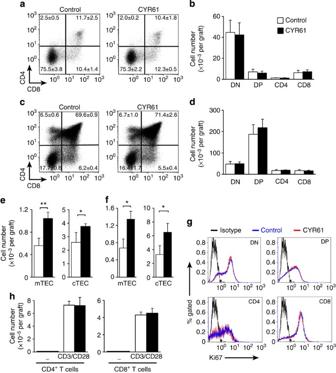Figure 6: CYR61 does not affect T-cell developmentper se. (a–f) Fetal thymus (FTOC) were cultured in the presence of CYR61-Fc (5 μg ml−1) for 2 days (a,b,e) or 6 days (c,d,f). Flow cytometry analysis of CD4/CD8 distribution (a,c) and thymocyte subset number (b,d) and TEC number (e,f). Data ±s.e.m. are representative of three independent experiments. *P≤0.05; **P≤0.01 (two-tailed unpaired Student’st-test). (g) Proliferative state of thymocytes in FTOC cultured in the presence of CYR61-Fc (5 μg ml−1) for 6 days. Data ±s.e.m. are representative of two independent experiments (h) T-cell proliferation assay. Cells were stimulated in anti-CD3-coated plates with anti-CD28 antibodies in presence of CYR61-Fc (5 μg ml−1) or Fc molecule for 72 h. Data are the mean of three experiments ±s.e.m. Figure 6: CYR61 does not affect T-cell development per se . ( a – f ) Fetal thymus (FTOC) were cultured in the presence of CYR61-Fc (5 μg ml −1 ) for 2 days ( a , b , e ) or 6 days ( c , d , f ). Flow cytometry analysis of CD4/CD8 distribution ( a , c ) and thymocyte subset number ( b , d ) and TEC number ( e , f ). Data ±s.e.m. are representative of three independent experiments. * P ≤0.05; ** P ≤0.01 (two-tailed unpaired Student’s t -test). ( g ) Proliferative state of thymocytes in FTOC cultured in the presence of CYR61-Fc (5 μg ml −1 ) for 6 days. Data ±s.e.m. are representative of two independent experiments ( h ) T-cell proliferation assay. Cells were stimulated in anti-CD3-coated plates with anti-CD28 antibodies in presence of CYR61-Fc (5 μg ml −1 ) or Fc molecule for 72 h. Data are the mean of three experiments ±s.e.m. Full size image The proliferative state of thymocytes after 6 days of CYR61 treatment was similar to that of controls as determined by Ki67 staining ( Fig. 6g ). Finally, presence of CYR61 during the T-cell proliferation assay using CD3/CD28 stimulation CYR61 did not further enhance T-cell proliferation or survival ( Fig. 6h ). These results show that starting with an equal number of progenitors, CYR61 treatment is not able to increase the production or promote the proliferation of T cells. Thus, a direct effect of CYR61 on thymocyte development can be excluded. CYR61 increases the hosting capacity for progenitors We then assessed the capacity of control lobes and CYR61-overexpressing lobes to import circulating progenitors with short-term homing assays [36] . WT-C57BL6 mice were transplanted under the renal capsule with control lobes in one kidney and CYR61 lobes in the other kidney ( Supplementary Fig. S7a ). Three weeks later, CFSE-labelled WT-bone marrow cells were injected i.v. After 48 h, thymic receptivity of grafted lobes was determined by counting the number of recruited Lin neg CFSE + cells ( Fig. 7a ) and Lin + CFSE + cells ( Fig. 7b ). We observed that the hosting capacity of expanded CYR61 lobes of precursors was significantly improved compared with control lobes ( Fig. 7a ). It should be noticed that increased receptivity of CYR61 lobes was not specific to precursor cells, as evidenced by the higher number of recruited Lin + CFSE + cells ( Fig. 7b ). 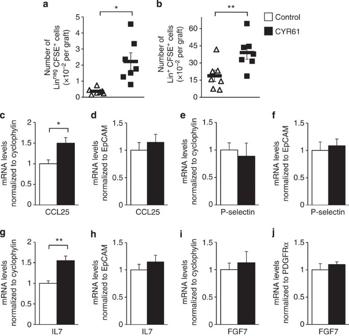Figure 7: CYR61 increases the hosting capacity of thymic lobes for circulating progenitors. (a,b) Three weeks after engraftment of CYR61 lobes and control lobes, CFSE-labelled WT-bone marrow cells were injected i.v. After 48 h, grafts were analysed for recruited LinnegCFSE+cells (a) and for Lin+CFSE+cells (b). Lin:B220, CD11c, CD11b, CD19, CD3, CD4, CD8, Ly6G, PDCA1, NK1.1, EpCAM. Results from two independent experiments are pooled (n=7). *P≤0.05; **P≤0.01 (paired Student’st-test). (c–j) FTOC were cultured in the presence of CYR61-Fc (5 μg ml−1) for 6 days. mRNA levels of CCL25 (c,d), P-selectin (e,f), IL7 (g,h) and FGF7 (i,j) were analysed by qPCR. Data±s.e.m. are representative of two independent experiments. *P≤0.05; **P≤0.01 (two-tailed unpaired Student’st-test). Figure 7: CYR61 increases the hosting capacity of thymic lobes for circulating progenitors. ( a , b ) Three weeks after engraftment of CYR61 lobes and control lobes, CFSE-labelled WT-bone marrow cells were injected i.v. After 48 h, grafts were analysed for recruited Lin neg CFSE + cells ( a ) and for Lin + CFSE + cells ( b ). Lin:B220, CD11c, CD11b, CD19, CD3, CD4, CD8, Ly6G, PDCA1, NK1.1, EpCAM. Results from two independent experiments are pooled ( n =7). * P ≤0.05; ** P ≤0.01 (paired Student’s t -test). ( c – j ) FTOC were cultured in the presence of CYR61-Fc (5 μg ml −1 ) for 6 days. mRNA levels of CCL25 ( c , d ), P-selectin ( e , f ), IL7 ( g , h ) and FGF7 ( i , j ) were analysed by qPCR. Data±s.e.m. are representative of two independent experiments. * P ≤0.05; ** P ≤0.01 (two-tailed unpaired Student’s t -test). Full size image The difference of recruitment of progenitors into CYR61 lobes can result from a passive (increased available space) or active process (increased chemokine production). Homing of progenitors is dependent on chemokines and cell adhesion molecules such as CCL25 and P-selectin [3] , [36] . FTOC treated with CYR61 for 6 days were analysed for expression of CCL25 and P-selectin. Overall CCL25 content in CYR61 lobes was increased compared with controls ( Fig. 7c ). This was an expected result because CYR61 treatment increases the number of TEC ( Figs 3a,b and 6e,f , Supplementary Fig. S7b ). After normalizing CCL25 levels to EpCAM, we observed no effect of CYR61 treatment on CCL25 expression ( Fig. 7d ). No difference was obtained for P-selectin ( Fig. 7e,f ). We conclude that the difference in the recruitment of progenitors into CYR61 lobes is passive. Other thymopoietic factors, such as IL7 and FGF7, were neither modified by CYR61 ( Fig. 7g–j ). These results show that CYR61 expands thymic stroma, thus improving available space in CYR61 lobes for hosting circulating progenitors. In addition, CYR61 is not able to directly promote the development of thymocytes. The generation of a self-tolerant T-cell repertoire is an intricate process. Progenitors recruited from the blood embrace the T-cell lineage fate within specific microenvironments created by stromal cells such as TEC [3] , [5] . Unfortunately, age-associated involution or atrophy of the thymus resulting from infection, chemotherapy or radiation all damage thymic architecture. This results in a decrease in TEC number and impairment of T-cell development, resulting in alteration of the T-cell repertoire and enhanced susceptibility to infections [6] . Therefore, unravelling the mechanisms mediating thymic stroma development is required for the development of therapies aimed at maintaining thymus function [6] . In this context, KGF administration was reported to enhance thymic recovery after irradiation and dexamethasone treatment [8] and to expand mTEC in Rag2 −/− mice [37] . Also, IL-22 administration accelerates the recovery of epithelial microenvironment after total body irradiation [9] , and miR-29a protects thymic epithelium from inappropriate infection-associated involution [38] . Finally, suppression of inflammasome-dependent caspase-1 activation decreases age-associated thymic involution by TEC and T-cell progenitors [39] . Matricellular CYR61 has been studied in cancer. Its binding to cell-surface integrins promotes cancer cell proliferation and metastasis. Notably, overexpression of CYR61 in breast, prostate or ovarian cancer cells enhances tumour growth [21] , [22] , [40] , whereas CYR61 silencing in pancreatic and prostate cancer cells decreases tumour growth [22] , [23] . Finally, recombinant CYR61 treatment accelerates repair of epithelium in vitro in a model of inflammatory lung epithelium injury [41] . As thymocytes and TEC undergo intense proliferation and apoptosis, we investigated whether matricellular CYR61 could improve TEC status and thymocyte development. Our findings demonstrate a beneficial impact of CYR61 treatment on progenitor handling and thymic output. Specifically, CYR61 induced the proliferation of TEC and expansion of thymic stroma, thereby increasing available space for the recruitment of circulating cells to then embrace normal T-cell development. Consequently, thymic output is improved ( Fig. 8 ). Our results provide evidence that modest overexpression of CYR61 efficiently expands the epithelial compartment. This represents a novel approach for improving or restoring immune competence. We propose CYR61 as an adjunctive treatment to thymus transplantation, which was performed successfully in patients with complete DiGeorge syndrome [34] or deficient for FoxN1 (ref. 35 ), and that restored T-cell production and function. Interestingly, CYR61 gene transfer has been used previously for therapeutic angiogenesis in models of lower-limb ischaemia [42] , ischaemic retinopathy [43] and experimental autoimmune myocarditis [44] . 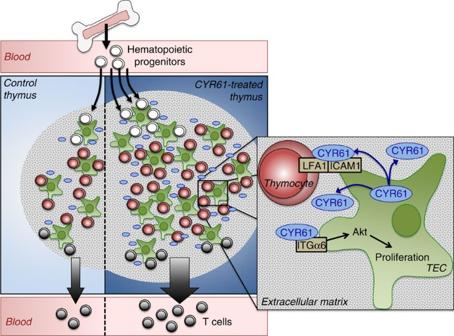Figure 8: CYR61-induced thymic stroma expansion increases thymic output. Matricellular CYR61 increases TEC proliferation and the size of the thymus. Expanded thymic stroma offers increased available space for the recruitment of circulating progenitors, which embrace normal T-cell development. Consequently, thymic output is improved. Figure 8: CYR61-induced thymic stroma expansion increases thymic output. Matricellular CYR61 increases TEC proliferation and the size of the thymus. Expanded thymic stroma offers increased available space for the recruitment of circulating progenitors, which embrace normal T-cell development. Consequently, thymic output is improved. Full size image Homing of circulating progenitors to the thymus is a tightly controlled process, which maintains continuous T-cell output without overgrowth of the thymus. Strikingly, this process is restricted by competition for limited stromal niches that provide important survival and differentiation factors [45] . Niche occupancy itself regulates the periodicity of expression of cell adhesion molecules and chemokines such as P-selectin and CCL25 in the thymus at steady state for progenitor importation [36] . A second level of control comes from the pool of peripheral lymphocytes that influence thymic P-selectin and CCL25 levels under acute conditions [36] . CYR61-overexpressing lobes exhibit increased thymic stromal size and receptivity for progenitor and Lin + cells without affecting relative CCL25 production. Therefore, our results can be explained by an increased number of niches in CYR61 lobes available for circulating progenitors. T-cell development is compartmentalized and dependent on adhesion events between maturing thymocytes and TEC. Although cell migration is guided by chemokine gradients, the ECM provides a structural support for cell migration and adhesion [10] , [46] . Hence, fibronectin and laminin produced by TEC favour thymocyte–TEC interactions as well as thymocyte migration through the thymus by binding to α4β1, α5β1 and α6β1 (refs 10 , 47 ). CYR61 is likely at the core of such interactions because it is known to bind to and thereby connect integrin α6 and ECM components (laminin, fibronectin and collagen) [14] . Here we show that CYR61 supports the adhesion of thymocytes to TEC through binding to LFA1 and ICAM1 or integrin α6 (ref. 47 ). CYR61 has also been reported to promote the adhesion and transendothelial migration of circulating hematopoietic CD34 + precursors [16] , as well as the migration of PBMC [20] . However, we did not observe chemotactic activity of CYR61 on developing thymocytes in similar transwell experiments. Integrin α6 is a target of CYR61 and responsible for its regulatory functions on cell adhesion, migration, senescence, apoptosis [14] and notably proliferation [27] . TEC adhesion, spreading and proliferation can be enhanced through activation of integrin α6 (ref. 47 ). Therefore, CYR61-mediated TEC proliferation likely results from binding to integrin α6. We did not observe any effect of CYR61 on thymocyte proliferation, in agreement with a previous study performed in our laboratory showing that blocking integrin α6 in FTOC did not influence T-cell development and proliferation [48] . CYR61-induced TEC proliferation was independent of thymocytes and was associated with the activation of the Akt signalling pathway. This is in accordance with previous studies showing that a reduced activity of Akt in TEC was responsible for altered thymic architecture and early involution [30] , as well as defects of keratinocyte proliferation [28] , [29] . Moreover, Akt was recently shown to be a target of CYR61 in lung epithelial cells [49] but also in PBMC, ovarian cancer, gastric cancer, cardiomyocytes and fibroblast-like synoviocytes [20] , [50] , [51] , [52] . Although, inhibition of Akt with MK2206 suppressed the proliferative effect of CYR61 on TEC, it also affected normal TEC homoeostasis. The effect of CYR61 on TEC occurred rapidly within 2 days in FTOC. The difference did not further increase significantly after 6 days, suggesting that recombinant CYR61 was no more active in culture. This loss of activity implicates that in vivo treatment with CYR61 protein for thymic involution for instance would require repeated protein administration or in situ delivery. Alternatively, thymic lobes may have reached a critical mass in vitro , avoiding any further growth. It should also be noticed that only the number of TEC were increased following CYR61 treatment in vitro and not other stromal cells such as endothelial cells. Therefore, CYR61 effects are mediated directly on TEC and not indirectly through improvement of angiogenesis, for instance. Thymus, lymph nodes, spleen and bone marrow share similarities with respect to their stromal cell-based architecture [53] , [54] . Therefore, our results on thymic stroma expansion by CYR61 offers new therapeutic perspectives and pave the way for studies on the developmental and functional implications of CYR61 in the immune response. Mice Mice were housed under specific pathogen-free conditions. Male C57BL6 nude mice (B6.Cg/NTac- Foxn1 nu NE10) were purchased from Taconic and were 8-weeks old on the day of engraftment. Male 6–8-week-old C57BL6 WT mice were from the CMU animal facility or purchased from Charles River. Pregnant C57BL6 WT mice were purchased from Charles River. All animal procedures were performed in accordance with the Institutional Ethical Committee of Animal Care in Geneva, Switzerland and the Cantonal Veterinary Office. Antibodies and proteins Control sheep Ig, polyclonal sheep anti-mouse CYR61 antibody (1/1000), recombinant human CYR61-Fc and Fc molecules were from R&D Systems. DyLight488-goat and DyLight650-goat anti-human Ig polyclonal antibody (1/1000) were from Abcam. A list of the other used antibodies is provided in Supplementary Table S1 . Quantitative RT–PCR Total RNA was prepared with TRIzol (Invitrogen). cDNA was synthesized with random hexamers and Superscript II RT (Invitrogen). qPCR was performed with iCycler iQ RT–PCR Detection System and iQ SYBR green Supermix (Bio-Rad). Results were quantified using a standard curve generated with serial dilutions of a reference cDNA. The list of the used primers is provided in Supplementary Table S2 . For CYR61 mRNA expression experiments, thymic populations were sorted on a MoFlow Astrios or an Aria Cell sorter. Purity of thymocytes was 99%. Purity of the other stromal populations was >85%. Immunostaining Thymi of 6–8-week-old mice were embedded in OCT (Sakura Finetek). Sections (20 μm) were fixed with 4% paraformaldehyde. Antibodies and secondary reagents were diluted in 0.1 M Tris (pH7.4) containing 5% of donkey serum (Jackson Immuno Research). Sections were counterstained with DAPI and mounted with Mowiol (Calbiochem). Images were acquired with a Zeiss LSM 510Meta confocal microscope (BioImaging Facility in CMU) and analysed with ImageJ software. Western blot Whole-cell extracts were obtained by cell lysis with 4 × Laemmli buffer. Extracts were loaded onto polyacrylamide gels, separated by electrophoresis and transferred onto Hybond–ECL membranes. Signal was generated with ECLPlus (Amersham). Chemiluminescence was recorded with LAS4000 (Fujifilm). Bands were quantified with Gel Analyzer tool in ImageJ. FTOC 2DG-FTOC and cell culture Thymic lobes isolated from 15.5-day embryos were cultured on Isopore membrane filters (Millipore) laid on gauze sponge in DMEM with 10% FCS, 2 mM Gln, 100 U ml −1 penicillin and streptomycin at 37 °C in a humidified atmosphere with 7% CO 2 for 2 or 6 days in the presence or absence of CYR61 (5 μg ml −1 ; 75.5 μM). For depletion of thymocytes, thymic lobes were cultured for 5 days with 1.35 mM 2′-deoxyguanosine (2DG; Sigma-Aldrich). After washing, lobes were further cultured for 4 days in presence of CYR61. Each experiment contained 4–8 lobes. Recombinant CYR61-Fc and Fc molecule were added on the first day of culture. IT76M1 cells were obtained from Dr P. Itoh (Japan) and initially developed from primary cultures of thymic stromal cells from Balb/c mice. IT76M1 were cultured in RPMI1640 with 10% heat-inactivated FCS, 2 mM Gln, 1 mM sodium pyruvate, 1% nonessential amino acids, 0,05 mM 2-mercaptoethanol, 100 U ml −1 penicillin and streptomycin at 37 °C in humidified atmosphere with 7% CO 2 . For signalling experiments, IT76M1 were cultured overnight in 5% FCS then cultured in medium supplemented with 1% FCS for 4 h. Kinetics were performed by adding CYR61 (5 μg ml −1 ) to the medium for the indicated times. Flow cytometry Labelling was performed in staining buffer (PBS containing 0.5% BSA, 5 mM EDTA). Cells were acquired with a FACS Gallios (Beckman Coulter) at the Flow Cytometry Facility in CMU and analysed with Kaluza software (Beckman Coulter). Doublets were excluded. For intracellular CYR61 staining, single-cell suspensions from whole thymus were prepared by digestion in HBSS containing collagenase (Roche) and DNase I. Cell preparations were then depleted of CD45 + cells using anti-CD45 magnetic beads and autoMACS (Miltenyi Biotec). Intracellular staining was performed with BD Cytofix/Cytoperm (BDBiosciences) according to the manufacturer’s instructions. For CYR61 staining, donkey serum was used instead of BSA. The use of collagenase for sample preparation and the presence of EDTA in staining buffer abolished CYR61 binding to cell surface. Thus, CYR61 staining only corresponds to intracellular CYR61. In addition, surface labelling for CYR61 is provided in Supplementary Fig. S1b . CYR61 binding experiments by flow cytometry For primary TEC, single-cell suspensions from whole thymus were prepared by digestion in HBSS containing liberase (Roche) and DNase I. Cell preparations were depleted of unwanted cells using biotin-coupled anti-CD45, anti-CD11b, anti-CD11c, anti-CD4, anti-CD8, anti-CD3, anti-NK1.1, anti B220, anti-CD19, anti-TER119 antibodies and anti-biotin magnetic beads. Negative selection was performed on MACS LS columns (Miltenyi Biotec). Cells were incubated in RPMI 0.5% BSA without EDTA at 37 °C for 4 h to recover from digestion and purification before CYR61 binding assay. For thymocytes, thymi were mechanically dissociated on 70-μm cell strainers and cells were resuspended in RPMI without EDTA. IT76 were detached from culture plates using cell detachment buffer (Invitrogen). Cells were pre-incubated with control rabbit Ig or polyclonal rabbit antibodies against integrin α6, αL, αM or ICAM1 for 45 min at RT in RPMI without EDTA. Then, cells were treated with recombinant Fc (75.5 μM) or CYR61-Fc (1 μg ml −1 ; 75.5 μM) for 15 min at RT. CYR61-Fc binding was detected using an AF488-coupled anti-human Fc antibody (Jackson Immuno Research). After washing in RPMI, binding was assessed by flow cytometry. In the case of primary TEC, we used recombinant Fc and CYR61-Fc that we directly coupled to DyLight 650 (Thermo Fischer). Thymocyte adhesion to TEC Thymocyte suspension was obtained by mechanical dissociation of thymi on 70-μm cell strainers. Thymocytes were CFSE-labelled and then added on IT76M1 cultured on μ-slide VI (Ibidi) pretreated with CYR61-Fc (5 μg ml −1 ; 75.5 μM) or Fc molecule (75.5 μM) for 60 min at 37 °C in DMEM. After 60 min at 37 °C, unbound thymocytes were washed away with fresh DMEM. Images were acquired with a Nikon A1r microscope (BioImaging Facility in CMU). Four independent experiments were performed. Adherent CFSE-cells were counted with Cell Counter plugin in ImageJ. T-cell proliferation assay Ninety six well plates were coated or not overnight at 4 °C with anti-CD3 antibody diluted in PBS (2 μg ml −1 ). Splenic CD4 + and CD8 + T cells were purified by positive selection and cultured in the presence or absence of anti-CD28 antibody (2 μg ml −1 ) in RPMI1640 with 20% heat-inactivated FCS, 2 mM Gln, 0.05 mM 2-mercaptoethanol, 100 U ml −1 penicillin and streptomycin at 37 °C. After 72 h, cells were counted with a Countess Automated Cell Counter (Invitrogen). In Fig. 6h , cells were cultured with CYR61 (5 μg ml −1 ; 75.5 μM) or Fc molecule (75.5 μM). Chemotaxis assay Effect of CYR61 on the migratory ability of thymocytes was assessed using 5-μm pore-size transwells (Costar). Thymocytes (2.5 × 10 6 ) were added in the upper chamber in RPMI1640, 0.5% BSA in the presence of CYR61-Fc (5 μg ml −1 ; 75.5 μM) or Fc molecule (75.5 μM). The lower chamber contained RPMI1640, 0.5% BSA with CYR61-Fc (5 μg ml −1 ; 75.5 μM) or Fc molecule (75.5 μM). After 3 h, percentage of input Lin neg (B220, CD11c, CD11b, CD19, F4/80, Ly6G, PDCA1, NK1.1, EpCAM) cells recovered in the lower compartment were determined by analysis with FACS Gallios. Lentiviral transduction of thymic lobes Mouse Cyr61 cDNA was subcloned from the pYX-Asc vector (Invitrogen) into the lentiviral pWPI vector containing an IRES-GFP sequence under the control of EF1α promoter. Recombinant lentiviruses were produced by co-transfecting 293T cells [55] . 2DG-treated lobes were cultured for 24 h in virus-containing medium, 50 μl being regularly added onto lobes. After 24 h, medium was replaced by fresh virus-containing medium for an additional 24 h. Lobes were further cultured for 3 days in normal medium. Thymic graft For thymic output experiments, six pieces of thymic lobes were grafted under the renal capsule of 8-week-old C57BL6 nude mice [56] . For short-term homing experiments and TCR Vβ usage, two pieces of CYR61 lobes were grafted under the kidney capsule of 8-week-old C57BL6 mice. One kidney was grafted with control lobes and the other one with CYR61 lobes. Short-term homing experiments were adapted from Gossens et al . [36] Three weeks after transplantation, each mouse was i.v. injected with 30 × 10 6 CFSE-labelled WT-bone marrow cells (7.5 μM, 5 min at 37 °C). After 48 h, mice were killed and CFSE + cells recruited to control and CYR61 lobes were counted with a FACS Gallios. Lin was defined as B220, CD11c, CD11b, CD19, CD3, CD4, CD8, Ly6G, PDCA1, NK1.1, EpCAM. Serum Ig levels Microtiter plates (Nunc) were coated with serum from grafted mouse. Bound IgG was captured by HRP-labelled anti-mouse IgG antibody (Jackson Immuno Research), revealed with Substrate Reagent (R&D Systems) and stopped by the addition of 0.5 N HCl. Serum IgG levels were determined at 450–570 nm. How to cite this article: Emre, Y. et al . Thymic epithelial cell expansion through matricellular protein CYR61 boosts progenitor homing and T-cell output. Nat. Commun. 4:2842 doi: 10.1038/ncomms3842 (2013).